Ephrin-A5/EphA4 signalling controls specific afferent targeting to cochlear hair cells Hearing requires an optimal afferent innervation of sensory hair cells by spiral ganglion neurons in the cochlea. Here we report that complementary expression of ephrin-A5 in hair cells and EphA4 receptor among spiral ganglion neuron populations controls the targeting of type I and type II afferent fibres to inner and outer hair cells, respectively. In the absence of ephrin-A5 or EphA4 forward signalling, a subset of type I projections aberrantly overshoot the inner hair cell layer and invade the outer hair cell area. Lack of type I afferent synapses impairs neurotransmission from inner hair cells to the auditory nerve. By contrast, radial shift of type I projections coincides with a gain of presynaptic ribbons that could enhance the afferent signalling from outer hair cells. Ephexin-1, cofilin and myosin light chain kinase act downstream of EphA4 to induce type I spiral ganglion neuron growth cone collapse. Our findings constitute the first identification of an Eph/ephrin-mediated mutual repulsion mechanism responsible for specific sorting of auditory projections in the cochlea. Hearing requires an optimal innervation of sensory hair cells (HCs), which transduce the acoustic signal. HCs receive two different types of innervation: afferent innervation from spiral ganglion (SG) neurons (SGNs) [1] , [2] and efferent innervation from the superior olivary complex [2] , [3] , [4] . The primary afferent innervation includes two functionally distinct neuronal populations conveying sound information from the cochlea to the central nervous system. In the adult sensory epithelium, the organ of Corti (OC), each inner HC (IHC) connects over 10 type I SGNs (about 90–95% of the neuronal population) and represents the principal encoder of the auditory signal. By contrast, outer HCs (OHCs) display an ‘en passant’ innervation by type II SGNs (approximately 5–10% of the total neuronal population) (Fig. 7a). The function of these type II connections is still unclear, but they may monitor and regulate OHC gain. In rodents, the development of cochlear innervation starts at early embryonic stages and is completed by the end of the first postnatal week. This process is divided into three main phases: (a) neurite growth and extension of type I and type II afferents to HCs (before birth), (b) axon refinement and HC innervation (postnatal day 0; P0–P3) and (c) neurite retraction and synaptic pruning (P3–P6) [5] . Axon guidance depends on the motility of navigating growth cones that respond to nondiffusible extracellular matrix molecules, transmembrane proteins expressed in neighbouring cells and diffusible chemotropic agents released by the target epithelium. These cues successively exert either repulsive or attractive influences on outgrowing axons and finally give rise to accurate targeting of auditory projections [6] . Importantly, although the mechanisms required for axon guidance to the OC become better characterized, the molecules underlying the specific refinement of type I and type II afferents to respective HCs remain elusive. Among gene families that have been shown to regulate neurite guidance, ephrins and their Eph receptors are good candidates for patterning auditory neural connectivity. Ephrin-As and EphA receptors are often expressed in complementary gradients in target cells and projecting neurons, respectively [7] , [8] . Particularly, both in vitro and in vivo findings have shown that ephrin-A5 induces growth cone collapse and axon repulsion upon binding to EphA receptors, avoiding formation and stabilization of axon branching and arborization at inaccurate locations [9] . This large Eph family has been classified into two subclasses, EphA and EphB, according to their affinity for either glycosylphosphatidylinositol-anchored ephrin-A or transmembrane ephrin-B ligands [10] . Immunohistochemical studies previously suggested alternating expression patterns of ephrins and Eph receptors in the developing inner ear [11] , [12] . On the basis of their well-described role in topographic mapping in several parts of central and peripheral nervous systems, we suggested that ephrin/Eph genes control the proper patterning of radial SGN projections in the cochlea. Here we found that ephrin-A5 and EphA4, expressed, respectively, in OHCs and type I SGNs, display complementary expression profiles at perinatal stages. In the absence of ephrin-A5 or EphA4 forward signalling, a subset of type I projections aberrantly overshoot the IHC layer and invade the OHC area, thereby suggesting an Eph/ephrin-mediated mutual repulsion mechanism responsible for specific afferent targeting to cochlear HCs. Differential expressions of ephrin-A5 and EphA4 Among the ephrin ligand family, ephrin-A5 is most commonly involved in topographic map specification through graded expression in the target region [9] , [13] , [14] . We therefore examined the ephrin-A5 expression in HCs during the formation of radial afferent projections in the cochlea. Ephrin-A5 mRNA and protein are specifically detected in OHCs between E18 and P4 ( Fig. 1j–n and Supplementary Fig. S1a–c ), a period characterized by neurite refinement and HC innervation [7] . Surprisingly, ephrin-A5 is also expressed in a subset of type I SGNs ( Fig. 1j and Supplementary Fig. 1d–f ). This ephrin-A5 + SGN subpopulation reaches a peak at P0 ( Fig. 1u and Supplementary Fig. 1d,e ). During the same time window, EphA4 is widely expressed in SG cells, especially in βIII-tubulin + SGNs ( Fig. 1a and Supplementary Fig. S1g–l ). However, both transcript and EphA4 EGFP remain preferentially confined to type I SGNs. Indeed, peripherin + type II SGNs [15] are negative for EphA4 expression ( Fig. 1a ). Among Eph receptors (that is, EphAs and EphB2 (ref. 16 )) that interact with ephrin-A5, EphA4 is the only one exhibiting such striking expression pattern in the SG, distinguishing type I from type II SGNs. EphA4 EGFP is also detectable in fibres that are specifically retained to IHCs at P2 ( Fig. 1g ). Taken together, these results suggest that ephrin-A5 and EphA4 display matching complementary expression profiles at perinatal stages ( Fig. 1v ), consistent with a role in specific afferent targeting to HCs in the cochlea. 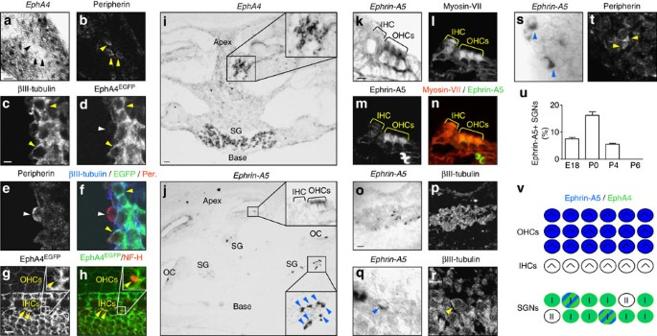Figure 1: Complementary expression patterns of ephrin-A5 and EphA4 in HCs and SGNs. (a,b) Confocal images of SG cells on transversal section of P0 cochlea processed for ISH withEphA4probe (a) and for peripherin immunostaining (b). Note that peripherin+type II SGNs (arrowheads inb) expressed lower levels ofEphA4as compared with peripherin−cells. (c–f) Triple immunolabeling on transversal section of SG from P0EphA4+/EGFPmouse showing that EphA4EGFPis expressed in SGNs (yellow arrowheads inc,d,f) but absent from peripherin+type II SGNs (white arrowhead ind–f). (g,h) Immunolabeling of whole-mount P2EphA4+/EGFPcochlea showing the presence of EGFP (arrowheads ing) in NF-H+fibres (arrowheads inh) retained at IHCs. ISH on transversal sections of P2 (i) and P0 (j) cochleae showing the expression ofEphA4(i) andephrin-A5(j) along the basal-to-apical axis of the cochlea. (k–n) ISH (k) and immunolabeling (l–n) on transversal section of a newborn mouse OC showing a prominent expression ofephrin-A5mRNA and protein in OHCs compared with IHC. (o–t) Confocal images of SG on transversal section of P0 cochlea processed for ISH withephrin-A5probe (o,q,s) and for βIII-tubulin (p,r) or peripherin immunostaining (t). Note thatephrin-A5is expressed in a subset of SGNs (blue arrowhead inq, yellow arrowhead inr) but is absent from peripherin+type II SGNs (blue arrowheads ins, yellow arrowheads int). (u) Quantification ofephrin-A5+SGNs across developmental stages. Thisephrin-A5+SGN subpopulation reaches a peak at P0. Data are presented as mean±s.e.m. (v) Schematic representation of ephrin-A5 (blue)/EphA4 (green) complementary expressions in HCs and SGNs in the perinatal cochlea. Note that ephrin-A5 expression likely overlaps EphA4 in a subset of type I SGNs. Scale bars in (a) represents 10 μm in (a,b), in (c), (g) and (k) 5 μm in (c–f,q–t), (g,h) and (k–n) respectively, in (i) and (o) 25 μm in (i,j) and (o,p) respectively. Figure 1: Complementary expression patterns of ephrin-A5 and EphA4 in HCs and SGNs. ( a , b ) Confocal images of SG cells on transversal section of P0 cochlea processed for ISH with EphA4 probe ( a ) and for peripherin immunostaining ( b ). Note that peripherin + type II SGNs (arrowheads in b ) expressed lower levels of EphA4 as compared with peripherin − cells. ( c – f ) Triple immunolabeling on transversal section of SG from P0 EphA4 +/EGFP mouse showing that EphA4 EGFP is expressed in SGNs (yellow arrowheads in c , d , f ) but absent from peripherin + type II SGNs (white arrowhead in d – f ). ( g , h ) Immunolabeling of whole-mount P2 EphA4 +/EGFP cochlea showing the presence of EGFP (arrowheads in g ) in NF-H + fibres (arrowheads in h ) retained at IHCs. ISH on transversal sections of P2 ( i ) and P0 ( j ) cochleae showing the expression of EphA4 ( i ) and ephrin-A5 ( j ) along the basal-to-apical axis of the cochlea. ( k – n ) ISH ( k ) and immunolabeling ( l – n ) on transversal section of a newborn mouse OC showing a prominent expression of ephrin-A5 mRNA and protein in OHCs compared with IHC. ( o – t ) Confocal images of SG on transversal section of P0 cochlea processed for ISH with ephrin-A5 probe ( o , q , s ) and for βIII-tubulin ( p , r ) or peripherin immunostaining ( t ). Note that ephrin-A5 is expressed in a subset of SGNs (blue arrowhead in q , yellow arrowhead in r ) but is absent from peripherin + type II SGNs (blue arrowheads in s , yellow arrowheads in t ). ( u ) Quantification of ephrin-A5 + SGNs across developmental stages. This ephrin-A5 + SGN subpopulation reaches a peak at P0. Data are presented as mean±s.e.m. ( v ) Schematic representation of ephrin-A5 (blue)/EphA4 (green) complementary expressions in HCs and SGNs in the perinatal cochlea. Note that ephrin-A5 expression likely overlaps EphA4 in a subset of type I SGNs. Scale bars in ( a ) represents 10 μm in ( a , b ), in ( c ), ( g ) and ( k ) 5 μm in ( c – f , q – t ), ( g , h ) and ( k – n ) respectively, in ( i ) and ( o ) 25 μm in ( i , j ) and ( o , p ) respectively. Full size image Mistargeting of afferent fibres to HCs in ephrin-A5 −/− cochlea To assess the role of ephrin-A5 in contributing to proper cochlear innervation, we performed neurofilament H (NF-H) and peripherin co-immunostaining on whole-mount post-hearing-onset (P14) cochleae [17] from wild type (WT) and ephrin-A5 −/− littermates [9] . Compared with the WT phenotype, a radial shift in innervation pattern from IHCs to OHCs is observed in ephrin-A5 −/− mice ( Fig. 2a–f ). In WT mice, most axons contacting OHCs belong to type II SGNs (NF-H + /peripherin + ) ( Fig. 2g ), as previously described [15] . By contrast, a large majority of fibres targeting the OHCs in ephrin-A5 −/− animals correspond to peripherin − ectopic innervation ( Fig. 2i ). Quantitative analysis revealed that the number of NF-H + /peripherin − projections to the OHC region is significantly increased in ephrin-A5 −/− P14 littermates ( Fig. 2u ). This suggests that loss of ephrin-A5 expression allowed a subset of type I SGNs to target the OHC layer instead of wiring with IHCs. In addition, although type II SGNs classically exhibit extensive arborization and innervate several OHCs in WT ( Fig. 2h ), they send shortened projections in ephrin-A5 −/− mice ( Fig. 2j ). The percentage of type II fibres whose length is < or > to 200 μm after entering the OC is, respectively, increased and decreased in ephrin-A5 −/− cochleae as compared with WT ( Fig. 2v ). This defect probably arises from axon competition induced by massive ectopic projections randomly invading the OHC area. Importantly, the number of IHC and OHC rows (1 and 3, respectively) and the number of total SGNs and peripherin + type II SGNs remain unchanged in the absence of ephrin-A5 ( Supplementary Figs S2 and S3a–f ). 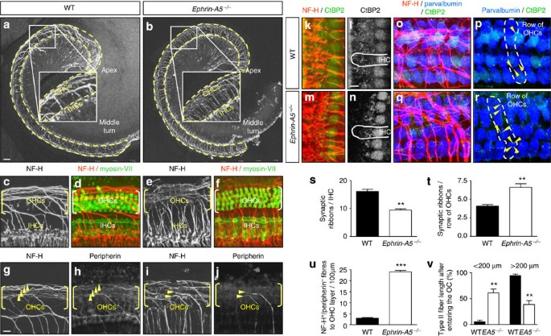Figure 2: Radial shift in afferent HC innervation pattern inephrin-A5−/−cochlea. (a–f) NF-H immunolabeling alone (a,b) or in combination with myosin-VII (c–f) of whole-mount cochleae from post-hearing-onset WT (a,c,d) andephrin-A5−/−(b,e,f) mice. Loss ofephrin-A5induces a radial shift in innervation pattern from the IHC to the OHC layers. The yellow dotted curve delimits the area of projections to OHCs. (g–j) Double immunolabeling for NF-H (g,i) and peripherin (h,j) on whole-mount cochleae from WT andephrin-A5−/−mice. (g,h) In WT mice, almost all projections to OHCs are identified as type II fibres (NF-H+/peripherin+) and exhibit extensive arborization (yellow arrowheads). (i,j) Inephrin-A5−/−mice, the OHC innervation is more abundant and largely attributable to ectopic NF-H+/peripherin−projections. In addition, type II afferents (peripherin+) show incomplete innervation (yellow arrowheads) compared with WT. Yellow brackets indicate the OHC area. (k–n) Double NF-H—CtBP2/RIBEYE immunolabeling focused on IHCs from WT (k,l) andephrin-A5−/−(m,n) mice. (o–r) Triple NF-H—parvalbumin—CtBP2/RIBEYE immunolabeling focused on OHCs from WT (o,p) andephrin-A5−/−(q,r) mice. (s) The number of synaptic ribbons per IHC is significantly reduced inephrin-A5−/−compared with WT mice (n=3 animals for both genotypes; **P<0.01). (t) The number of synaptic ribbons per row of OHCs is significantly increased inephrin-A5−/−compared with WT mice (n=3 animals for both genotypes; **P<0.01). (u) The number of NF-H+/peripherin−fibres targeting the OHC layer is significantly increased inephrin-A5−/−compared with WT mice (n=3 animals for both genotypes; ***P<0.001). (v) The percentage of type II fibres of which length is<or>to 200 μm after entering the OC is, respectively, significantly increased and decreased compared with WT (n=3 animals for both genotypes; **P<0.01). Statistical significance was determined using Student’st-test. Data are presented as mean±s.e.m. Scale bars in (a) represent 50 μm in (a,b) and 10 μm in (c–f), in (g) 10 μm in (g–j), in (l) 5 μm in (k–r), respectively. Figure 2: Radial shift in afferent HC innervation pattern in ephrin-A5 −/− cochlea. ( a – f ) NF-H immunolabeling alone ( a , b ) or in combination with myosin-VII ( c – f ) of whole-mount cochleae from post-hearing-onset WT ( a , c , d ) and ephrin-A5 −/− ( b , e , f ) mice. Loss of ephrin-A5 induces a radial shift in innervation pattern from the IHC to the OHC layers. The yellow dotted curve delimits the area of projections to OHCs. ( g – j ) Double immunolabeling for NF-H ( g , i ) and peripherin ( h , j ) on whole-mount cochleae from WT and ephrin-A5 −/− mice. ( g , h ) In WT mice, almost all projections to OHCs are identified as type II fibres (NF-H + /peripherin + ) and exhibit extensive arborization (yellow arrowheads). ( i , j ) In ephrin-A5 −/− mice, the OHC innervation is more abundant and largely attributable to ectopic NF-H + /peripherin − projections. In addition, type II afferents (peripherin + ) show incomplete innervation (yellow arrowheads) compared with WT. Yellow brackets indicate the OHC area. ( k – n ) Double NF-H—CtBP2/RIBEYE immunolabeling focused on IHCs from WT ( k , l ) and ephrin-A5 −/− ( m , n ) mice. ( o – r ) Triple NF-H—parvalbumin—CtBP2/RIBEYE immunolabeling focused on OHCs from WT ( o , p ) and ephrin-A5 −/− ( q , r ) mice. ( s ) The number of synaptic ribbons per IHC is significantly reduced in ephrin-A5 −/− compared with WT mice ( n =3 animals for both genotypes; ** P <0.01). ( t ) The number of synaptic ribbons per row of OHCs is significantly increased in ephrin-A5 −/− compared with WT mice ( n =3 animals for both genotypes; ** P <0.01). ( u ) The number of NF-H + /peripherin − fibres targeting the OHC layer is significantly increased in ephrin-A5 −/− compared with WT mice ( n =3 animals for both genotypes; *** P <0.001). ( v ) The percentage of type II fibres of which length is<or>to 200 μm after entering the OC is, respectively, significantly increased and decreased compared with WT ( n =3 animals for both genotypes; ** P <0.01). Statistical significance was determined using Student’s t -test. Data are presented as mean±s.e.m. Scale bars in ( a ) represent 50 μm in ( a , b ) and 10 μm in ( c – f ), in ( g ) 10 μm in ( g – j ), in ( l ) 5 μm in ( k – r ), respectively. Full size image Sensory synapses of the auditory system must faithfully encode a wide dynamic range of graded signals, and must be capable of sustained transmitter release over long periods of time. These properties require specialized structures called synaptic ribbons. These ribbons are electron-dense presynaptic specializations that tether synaptic vesicles, allowing rapid exocytosis and fast synaptic transmission [18] , [19] . The major structural component of synaptic ribbons identified so far is RIBEYE, a protein aggregate formed by a unique and ribbon-specific A domain, and a dimeric B domain identical to CtBP2, a transcriptional repressor protein [20] . In the mammalian cochlea, outside of the extreme apex, >95% of cochlear nerve fibres are unbranched, contacting a single IHC via a single terminal swelling, with a single active zone at which a single presynaptic ribbon is tethered to the IHC membrane [21] . Thus, ribbon quantifications provide an accurate metric of the IHC afferent innervation [22] . It has to be pointed out that CtBP2 + ribbons are not systematically coupled to NF-H + staining, because neurofilaments do not fill terminal axon swellings [22] . Consistent with the finding that some type I SGNs aberrantly project to the OHC region in ephrin-A5 −/− mice, mean counts revealed a significant decrease of presynaptic active zones per IHC in ephrin-A5 −/− compared with WT mice ( Fig. 2k–n ). We then wondered whether the lack of IHC afferent synapses in ephrin-A5 − / − cochlea coincides with a gain of OHC synaptic ribbons. Ribbon counts revealed a significant increase of presynaptic active zones per row of OHCs in ephrin-A5 −/− compared with WT mice ( Fig. 2o–r ). Combination of both results suggests that, in ephrin-A5 −/− mice, the radial shift of type I projections from IHC to OHC layers is accompanied by a similar radial displacement of presynaptic active zones. Ephrin-A5/EphA4 is required for SGN projection sorting When present in target cells, ephrin-A5 induces axon growth cone repulsion through activation of EphA receptors, avoiding propagation of ectopic projections in the region of expression [9] , [23] . To further understand the mechanism of axonal refinement in the OC occurring between P0 and P3, we considered using whole-mount cochleae from 2-day-old WT and ephrin-A5 −/− mice ( Fig. 3a ). At this stage, growing type I projections that have reached the first row of OHCs are progressively redirected to the basolateral region of IHCs [5] . In that respect, we observed that, in WT animals, most of the growing axons are stopped just beneath the first row of OHCs ( Fig. 3b ). By contrast, almost no refining fibres are distinguishable in the absence of ephrin-A5 . A huge amount of neurites, instead of being repulsed by ephrin-A5 + OHCs, abnormally overshoot the IHC layer and give rise to an aberrant OHC projection pattern ( Fig. 3c ). The proportion of fibres targeting the OHC layer is significantly higher in ephrin-A5 −/− compared with WT animals ( Fig. 3l ). 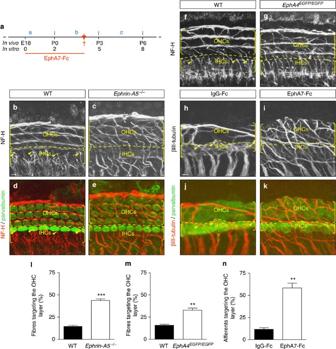Figure 3: Ephrin-A5/EphA4 forward signalling is required for the sorting of radial SGN projections. (a) Schematic representation ofin vivoandin vitroprotocols used to analyse cochlear innervation. (a) Type I and type II neurite extension to HCs (before birth), (b) neurite refinement and HC innervation (P0–P3) and (c) neurite retraction and synaptic pruning (P3–P6). WT andephrin-A5−/−mice were killed at P2 (red cross). Explants of OC and SG from E18 embryos were treatedin vitrowith EphA7-Fc during 4 days (red bar). (b–g) Immunolabeling for NF-H alone or in combination with parvalbumin of whole-mount cochlea from P2 WT,ephrin-A5−/−andEphA4EGFP/EGFPmice. (b,d,f) In WT condition, most growth cones (arrowheads) stop beneath the first row of OHCs (dotted line). Inephrin-A5−/−(c,e) orEphA4EGFP/EGFP(g) mice, almost no collapsed growth cones can be observed, whereas many fibres aberrantly invade the OHC layer. (h–k)In vitroorganotypic model using SG and OC cultured in the presence of control (IgG-Fc;h,j) or the soluble inhibitor EphA7-Fc (i,k) reagents. Double immunolabeling for βIII-tubulin and parvalbumin. (h,j) In the control condition, almost all afferent projections are retained to IHCs, and some stopping growth cones (arrowheads) can be observed at the limit between IHC and OHC layers (yellow dotted line). (i,k) When blocking endogenous ephrin-A5 signalling, a majority of fibres project to the OHC layer. (l,m) The proportion of fibres targeting the OHC region is significantly increased inephrin-A5−/−(l) andEphA4EGFP/EGFP(m) versus WT mice (n=3 animals for each genotype, **P<0.01, ***P<0.001). (n) The proportion of afferent fibres targeting the OHC region is significantly increased in EphA7-Fc versus IgG-Fc condition (n=3 independent experiments for both conditions; **P<0.01). Statistical significance was determined using Student’st-test. Data are presented as mean±s.e.m. Scale bars in (b) and (h) represent 5 μm in (b–g) and (h–k), respectively. Figure 3: Ephrin-A5/EphA4 forward signalling is required for the sorting of radial SGN projections. ( a ) Schematic representation of in vivo and in vitro protocols used to analyse cochlear innervation. ( a ) Type I and type II neurite extension to HCs (before birth), ( b ) neurite refinement and HC innervation (P0–P3) and ( c ) neurite retraction and synaptic pruning (P3–P6). WT and ephrin-A5 −/− mice were killed at P2 (red cross). Explants of OC and SG from E18 embryos were treated in vitro with EphA7-Fc during 4 days (red bar). ( b – g ) Immunolabeling for NF-H alone or in combination with parvalbumin of whole-mount cochlea from P2 WT, ephrin-A5 −/− and EphA4 EGFP/EGFP mice. ( b , d , f ) In WT condition, most growth cones (arrowheads) stop beneath the first row of OHCs (dotted line). In ephrin-A5 −/− ( c , e ) or EphA4 EGFP/EGFP ( g ) mice, almost no collapsed growth cones can be observed, whereas many fibres aberrantly invade the OHC layer. ( h – k ) In vitro organotypic model using SG and OC cultured in the presence of control (IgG-Fc; h , j ) or the soluble inhibitor EphA7-Fc ( i , k ) reagents. Double immunolabeling for βIII-tubulin and parvalbumin. ( h , j ) In the control condition, almost all afferent projections are retained to IHCs, and some stopping growth cones (arrowheads) can be observed at the limit between IHC and OHC layers (yellow dotted line). ( i , k ) When blocking endogenous ephrin-A5 signalling, a majority of fibres project to the OHC layer. ( l , m ) The proportion of fibres targeting the OHC region is significantly increased in ephrin-A5 −/− ( l ) and EphA4 EGFP/EGFP ( m ) versus WT mice ( n =3 animals for each genotype, ** P <0.01, *** P <0.001). ( n ) The proportion of afferent fibres targeting the OHC region is significantly increased in EphA7-Fc versus IgG-Fc condition ( n =3 independent experiments for both conditions; ** P <0.01). Statistical significance was determined using Student’s t -test. Data are presented as mean±s.e.m. Scale bars in ( b ) and ( h ) represent 5 μm in ( b – g ) and ( h – k ), respectively. Full size image To ascertain the requirement of ephrin-A5 in specific SGN afferent targeting to HCs, we used an organotypic assay, in which explants of OC and SG (devoid of efferent fibres from the brainstem) were isolated from E18 cochleae and cultured in order to examine the effect of acute ephrin-A5 signalling inhibition in vitro . To avoid any disruption with findings suggesting an EphA4-mediated axon guidance to the OC through binding to ephrin-B2 and -B3 (refs 24 , 25 ), we preferred to treat with soluble EphA7-Fc known to have a high affinity for ephrin-A5 [10] rather than with EphA4-Fc. Tissues were maintained for 4 days in culture to analyse the processes of selective neurite refinement and HC innervation ( Fig. 3a ). In the control condition (IgG-Fc), the majority of growing axons are ending at the IHC level ( Fig. 3h ). By contrast, when blocking ephrin-A5-binding sites, most fibres extend radially to the OHC area ( Fig. 3i ). The proportion of afferent fibres targeting the OHC layer is significantly higher in EphA7-Fc compared with the control condition ( Fig. 3n ) without affecting neuron survival ( Supplementary Fig. S3m,n,r ). Both control and EphA7-Fc culture conditions seem to faithfully reproduce the stage of neurite refinement to HCs observed at P2 in WT and ephrin-A5 −/− mice, respectively. These results confirm the involvement of ephrin-A5 in specific afferent targeting to HCs in the cochlea. In support of this finding, a neuronal tracing experiment revealed that ephrin-A5 − / − mice do not display any radial shift in efferent innervation pattern from IHCs to OHCs compared with WT animals ( Supplementary Fig. S4 ). Altogether, these results indicate that mistargeting of afferent fibres is the single cause of the radial shift in HC innervation pattern observed in ephrin-A5 − / − cochleae. To test whether EphA4 is the receptor through which ephrin-A5 induces sorting of SGN projections, we used a mouse line encoding an EphA4 forward signalling-deficient isoform [26] . The proportion of fibres targeting the OHC layer was found to be significantly higher in EphA4 EGFP/EGFP compared with WT animals both at P2 ( Fig. 3f ) and after hearing onset ( Fig. 4a–j ). Ribbon counts confirmed this radial shift from the IHC layer to the OHC layer in EphA4 EGFP/EGFP mice ( Fig. 4k–p ), whereas both βIII-tubulin + (type I and II) and peripherin + (type II) SGN survival remain unchanged ( Supplementary Fig. S3g-l ). In contrast, the percentage of type II fibres whose length is < or > to 200 μm after entering the OC is, respectively, increased and decreased in EphA4 EGFP/EGFP mice as compared with WT ( Fig. 4g–j ), suggesting a mechanism of axon competition. Mimicking the ephrin-A5 − / − phenotype, these results therefore suggest that EphA4 forward signalling is required for sorting of radial SGN projections. 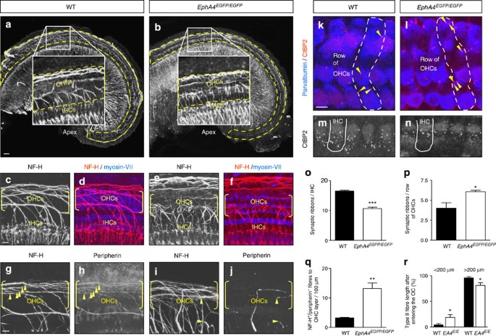Figure 4: Radial shift in HC afferent innervation pattern in post-hearing-onset EphA4 forward-signalling-deficient mice. (a–f) NF-H immunolabeling alone (a,b) or in combination with myosin-VII (c–f) of whole-mount cochleae from post-hearing-onset WT (a,c,d) andEphA4EGFP/EGFP(b,e,f) animals. Loss of EphA4 forward signalling induces a radial shift in innervation pattern from IHC to OHC layers. The yellow dotted curve delimits the area of projections to OHCs. (g–j) Double immunolabeling for NF-H (g,i) and peripherin (h,j) on whole-mount cochleae from WT andEphA4EGFP/EGFPmice. (g,h) In WT mice, almost all projections to OHCs are identified as type II fibres (NF-H+/peripherin+) and exhibit extensive arborization (yellow arrowheads). (i,j) In EphA4-knocking mice, the OHC innervation is more abundant and largely attributable to ectopic NF-H+/peripherin−projections. In addition, type II afferents (peripherin+) show incomplete innervation (yellow arrowheads) compared with WT. Yellow brackets indicate the OHC area. (k,l) Double parvalbumin—CtBP2/RIBEYE immunolabeling focused on OHCs from WT (k) andEphA4EGFP/EGFP(l) mice. (m,n) CtBP2/RIBEYE immunolabeling focused on IHCs from WT (m) andEphA4EGFP/EGFP(n) mice. (o) The number of synaptic ribbons per IHC is significantly reduced inephrin-A5−/−compared with WT mice (n=3 animals for both genotypes; ***P<0.001). (p) The number of synaptic ribbons per row of OHCs is significantly increased inEphA4EGFP/EGFPcompared with WT mice (n=3 animals for both genotypes; *P<0.05). (q) The number of NF-H+/peripherin−fibres targeting the OHC layer is significantly increased inEphA4EGFP/EGFPcompared with WT mice (n=3 animals for both genotypes; **P<0.01). (r) The percentage of type II fibres whose length is<or>to 200 μm after entering the OC is, respectively, significantly increased and decreased compared with WT (n=4 animals for both genotypes; *P<0.05). Statistical significance was determined using Student’st-test. Data are presented as mean±s.e.m. Scale bar in (a) represents 50 μm in (a,b), in (c) and (g) 10 μm in (c–f) and (g–j), respectively, in (k) 5 μm in (k–n). Figure 4: Radial shift in HC afferent innervation pattern in post-hearing-onset EphA4 forward-signalling-deficient mice. ( a – f ) NF-H immunolabeling alone ( a , b ) or in combination with myosin-VII ( c – f ) of whole-mount cochleae from post-hearing-onset WT ( a , c , d ) and EphA4 EGFP/EGFP ( b , e , f ) animals. Loss of EphA4 forward signalling induces a radial shift in innervation pattern from IHC to OHC layers. The yellow dotted curve delimits the area of projections to OHCs. ( g – j ) Double immunolabeling for NF-H ( g , i ) and peripherin ( h , j ) on whole-mount cochleae from WT and EphA4 EGFP/EGFP mice. ( g , h ) In WT mice, almost all projections to OHCs are identified as type II fibres (NF-H + /peripherin + ) and exhibit extensive arborization (yellow arrowheads). ( i , j ) In EphA4-knocking mice, the OHC innervation is more abundant and largely attributable to ectopic NF-H + /peripherin − projections. In addition, type II afferents (peripherin + ) show incomplete innervation (yellow arrowheads) compared with WT. Yellow brackets indicate the OHC area. ( k , l ) Double parvalbumin—CtBP2/RIBEYE immunolabeling focused on OHCs from WT ( k ) and EphA4 EGFP/EGFP ( l ) mice. ( m , n ) CtBP2/RIBEYE immunolabeling focused on IHCs from WT ( m ) and EphA4 EGFP/EGFP ( n ) mice. ( o ) The number of synaptic ribbons per IHC is significantly reduced in ephrin-A5 −/− compared with WT mice ( n =3 animals for both genotypes; *** P <0.001). ( p ) The number of synaptic ribbons per row of OHCs is significantly increased in EphA4 EGFP/EGFP compared with WT mice ( n =3 animals for both genotypes; * P <0.05). ( q ) The number of NF-H + /peripherin − fibres targeting the OHC layer is significantly increased in EphA4 EGFP/EGFP compared with WT mice ( n =3 animals for both genotypes; ** P <0.01). ( r ) The percentage of type II fibres whose length is<or>to 200 μm after entering the OC is, respectively, significantly increased and decreased compared with WT ( n =4 animals for both genotypes; * P <0.05). Statistical significance was determined using Student’s t -test. Data are presented as mean±s.e.m. Scale bar in ( a ) represents 50 μm in ( a , b ), in ( c ) and ( g ) 10 μm in ( c – f ) and ( g – j ), respectively, in ( k ) 5 μm in ( k – n ). Full size image Ephrin-A5/EphA4 induces type I SGN growth cone collapse To confirm the hypothesis that EphA4 is required for type I axon repulsion upon binding to ephrin-A5, we performed growth cone collapse assays, in which dissociated SGNs from newborn mouse cochleae are exposed to pre-clustered ephrin-A5. After treatment, the majority of SGN neurites undergo growth cone collapse, as revealed by the F-actin marker phalloidin ( Fig. 5b ). The size reduction of growth cones (compare Fig. 5a ) is correlated with phosphorylation of EphA4 on tyr-602 residue ( Fig. 5b ) [27] . By contrast, SGNs preferentially show large growth cones in the control condition, with no detectable EphA4 phopho-specific immunolabeling ( Fig. 5a ). Importantly, growth cones of peripherin + type II SGNs appear not sensitive to pre-clustered ephrin-A5, and remain similar to those found in the control condition ( Fig. 5f ). Quantitative analysis revealed that the proportion of type I growth cone collapse is significantly increased upon stimulation with ephrin-A5-Fc compared with the control condition ( Fig. 5q ). Such a result was confirmed using an in vitro stripe assay, in which a majority of SG growth cones avoid the ephrin-A5-Fc-containing stripes ( Supplementary Fig. 5 ). On the contrary, type I SGN growth cones from EphA4 EGFP/EGFP mice, in which EGFP is expressed, do not collapse in the presence of ephrin-A5-Fc ( Fig. 5g ). These results therefore suggest that ephrin-A5 selectively induces growth cone collapse on type I SGNs through specific activation of EphA4. 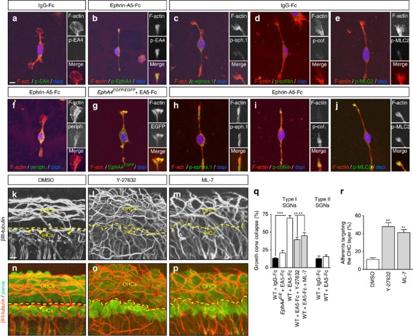Figure 5: Ephrin-A5 induces growth cone collapse on type I SGNs through activation of EphA4. (a,b,f,g) Representative examples ofin vitrogrowth cone collapse assay on dissociated SGNs from newborn mice using control IgG-Fc or pre-clustered ephrin-A5-Fc. (a) In the control condition, SGNs show a large growth cone with no sign of EphA4 phosphorylation. (b) Upon incubation with pre-clustered ephrin-A5-Fc, F-actin marker tetramethyl rhodamine isothiocyanate-phalloidin (red) reveals severe growth cone collapse simultaneously co-localized with EphA4 phospho-specific (tyr-602) immunolabeling. (f) Growth cones of type II SGNs (peripherin+, green) are not sensitive to clustered ephrin-A5, and their structure remains similar to those observed in the control condition. (g) Type I SGN growth cones fromEphA4EGFP/EGFPmice, in which EGFP is expressed, do not collapse in the presence of ephrin-A5-Fc. (c–e,h–j) Signalling proteins downstream of EphA4 activation. Ephrin-A5-induced growth cone collapse coincides with phosphorylation of ephexin-1 (h), cofilin (i) and myosin light chain-2 (MLC-2) (j) compared with control condition (c,d,e). (k–p)In vitroorganotypic model using SG and OC cultured in the presence of dimethylsulphoxide (k,n), Y-27632 (l,o) or ML-7 (m,p). (k,n) Under control conditions, almost all afferent fibres are retained to IHCs and some stopping fibres (arrowheads) can be observed at the limit between IHC and OHC layers (yellow dotted line). When blocking endogenous ROCK (l,o) or MLCK (m,p) signalling pathways, a majority of fibres project to the OHC layer. (q) The proportion of type I growth cone collapse is significantly increased upon stimulation with ephrin-A5-Fc compared with the control condition, but not when type I SGNs lack EphA4 forward signalling. This effect is significantly rescued by pre-treatment with either Y-27632 or ML-7. By contrast, the proportion of type II growth cone collapse is not increased upon stimulation with ephrin-A5-Fc compared with the control condition.n=3 independent experiments for each condition. **P<0.01, ***P<0.001. (r) The percentage of afferent fibres targeting the OHC layer is significantly increased in the presence of either Y-27632 or ML-7 inhibitors.n=3 independent experiments for each condition. **P<0.01 Statistical significance was determined using one-way ANOVA test followed by a Dunnett’s post-test. Data are presented as mean±s.e.m. Scale bars in (a) and (k) represent 5 μm in (a-j) and (k–p), respectively. Figure 5: Ephrin-A5 induces growth cone collapse on type I SGNs through activation of EphA4. ( a , b , f , g ) Representative examples of in vitro growth cone collapse assay on dissociated SGNs from newborn mice using control IgG-Fc or pre-clustered ephrin-A5-Fc. ( a ) In the control condition, SGNs show a large growth cone with no sign of EphA4 phosphorylation. ( b ) Upon incubation with pre-clustered ephrin-A5-Fc, F-actin marker tetramethyl rhodamine isothiocyanate-phalloidin (red) reveals severe growth cone collapse simultaneously co-localized with EphA4 phospho-specific (tyr-602) immunolabeling. ( f ) Growth cones of type II SGNs (peripherin + , green) are not sensitive to clustered ephrin-A5, and their structure remains similar to those observed in the control condition. ( g ) Type I SGN growth cones from EphA4 EGFP/EGFP mice, in which EGFP is expressed, do not collapse in the presence of ephrin-A5-Fc. ( c – e , h – j ) Signalling proteins downstream of EphA4 activation. Ephrin-A5-induced growth cone collapse coincides with phosphorylation of ephexin-1 ( h ), cofilin ( i ) and myosin light chain-2 (MLC-2) ( j ) compared with control condition ( c , d , e ). ( k – p ) In vitro organotypic model using SG and OC cultured in the presence of dimethylsulphoxide ( k , n ), Y-27632 ( l , o ) or ML-7 ( m , p ). ( k , n ) Under control conditions, almost all afferent fibres are retained to IHCs and some stopping fibres (arrowheads) can be observed at the limit between IHC and OHC layers (yellow dotted line). When blocking endogenous ROCK ( l , o ) or MLCK ( m , p ) signalling pathways, a majority of fibres project to the OHC layer. ( q ) The proportion of type I growth cone collapse is significantly increased upon stimulation with ephrin-A5-Fc compared with the control condition, but not when type I SGNs lack EphA4 forward signalling. This effect is significantly rescued by pre-treatment with either Y-27632 or ML-7. By contrast, the proportion of type II growth cone collapse is not increased upon stimulation with ephrin-A5-Fc compared with the control condition. n =3 independent experiments for each condition. ** P <0.01, *** P <0.001. ( r ) The percentage of afferent fibres targeting the OHC layer is significantly increased in the presence of either Y-27632 or ML-7 inhibitors. n =3 independent experiments for each condition. ** P <0.01 Statistical significance was determined using one-way ANOVA test followed by a Dunnett’s post-test. Data are presented as mean±s.e.m. Scale bars in ( a ) and ( k ) represent 5 μm in ( a - j ) and ( k – p ), respectively. Full size image We then tested whether the RhoA-associated kinase (ROCK)/myosin light chain kinase (MLCK) signalling pathway is involved in ephrin-A5-induced growth cone collapse, as previously shown in retinal ganglion cell [28] and hippocampal explant cultures [29] , respectively. Incubation of either p160 ROCK-specific inhibitor Y-27632 or MLCK inhibitor ML-7 in primary culture of SGNs result in a significant rescue of ephrin-A5-induced growth cone collapse ( Fig. 5q ). These results were confirmed in organotypic culture assay. Blocking either ROCK or MLCK results in a radial shift of afferent innervation pattern from IHC to OHC layers as compared with control (dimethylsulphoxide) condition ( Fig. 5k–p ), without affecting neuron survival ( Supplementary Fig. S3o–r ). In addition, we found that growth cone collapse coincides with phosphorylation of three potential downstream signalling proteins of EphA4: the guanine nucleotide exchange factor ephexin-1 [30] , the actin-depolymerizing and -severing factor cofilin-1 [31] and the ATP-dependent motor protein myosin-2 (responsible for actin-based motility) [32] ( Fig. 5h , respectively). These findings support a requirement of the RhoA-ROCK/cofilin/MLCK signalling pathway downstream of EphA4 receptor activation by ephrin-A5 (Fig. 7d). Ephrin-A5 is required for optimal IHC neurotransmission To assess the hearing function when ephrin-A5 is missing, we performed auditory brainstem response (ABR) recordings on 3-month-old WT and ephrin-A5 −/− mice, as we found that radial shift in HC innervation pattern is conserved until adulthood (as shown in the apical turn, Supplementary Fig. S6 ). ABR measurements were obtained using click stimuli. Hearing thresholds remained similar for both genotypes ( Fig. 6a ). However, ABR amplitudes to suprathreshold click stimuli were altered in ephrin-A5 −/− animals. In particular, ABR peak 1 amplitude reflecting the summed activity of cochlear afferents [33] , [34] is significantly decreased at several intensity levels and, on average, is 40% smaller in mice lacking ephrin-A5 ( Fig. 6b ). This deficient neurotransmission probably arises from reduced number of IHC afferent connections by type I SGNs caused by partial mistargeting of type I projections to OHCs ( Fig. 2 and Supplementary Fig. S6 ). 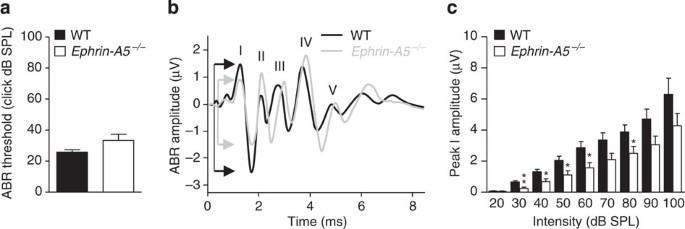Figure 6: Ephrin-A5 is required for optimal neurotransmission from IHCs to the auditory nerve. (a) Hearing thresholds are similar in both WT andephrin-A5−/−mice. ABR measurements were established using click stimuli. (b) ABR waveforms fromephrin-A5−/−(grey) exhibit decreased peak I amplitude compared with WT (black) mice. Peak II is generated by the central portion of VIIIth cranial nerve; Peak III by the cochlear nucleus; Peak IV by the superior olivary complex/lateral lemniscus; Peak V by the lateral lemniscus/inferior colliculus. (c) Peak I amplitude is significantly reduced when using 30, 40, 50, 60 and 80 dB SPL stimulation and, on average, is 40% smaller inephrin-A5−/−mice.n=12 animals for both genotypes. *P<0.05, **P<0.01. Statistical significance was determined using Student’st-test. Data are presented as mean±s.e.m. Figure 6: Ephrin-A5 is required for optimal neurotransmission from IHCs to the auditory nerve. ( a ) Hearing thresholds are similar in both WT and ephrin-A5 −/− mice. ABR measurements were established using click stimuli. ( b ) ABR waveforms from ephrin-A5 −/− (grey) exhibit decreased peak I amplitude compared with WT (black) mice. Peak II is generated by the central portion of VIIIth cranial nerve; Peak III by the cochlear nucleus; Peak IV by the superior olivary complex/lateral lemniscus; Peak V by the lateral lemniscus/inferior colliculus. ( c ) Peak I amplitude is significantly reduced when using 30, 40, 50, 60 and 80 dB SPL stimulation and, on average, is 40% smaller in ephrin-A5 −/− mice. n =12 animals for both genotypes. * P <0.05, ** P <0.01. Statistical significance was determined using Student’s t -test. Data are presented as mean±s.e.m. Full size image In the mid 1990s, it was suggested that brain-derived neurotrophic factor and neurotrophin-3 specifically support the innervation of OHCs and IHCs through activation of trkB or trkC receptors on type II and type I SGNs, respectively [35] . However, further studies revealed that, even if neurotrophins via trk receptors clearly promote SGN survival and fibre outgrowth during development, these molecules fail to explain by themselves the formation of proper afferent connections between HCs and SGNs [36] . In this study, we provide a model describing how type I and type II SGNs specifically innervate IHCs and OHCs, respectively. This mechanism involves complementary and specific spatio-temporal expressions of ephrin-A5 in OHCs and EphA4 in type I SGNs throughout the perinatal period of axonal refinement leading to HC innervation ( Fig. 1 ) [5] . Analysis of ephrin-A5 −/− mice suggests that a subset of type I SGNs overshoot the IHCs and abnormally project into the OHC region, adopting consequently the behaviour of type II innervation ( Fig. 7b ). This phenotype was reproduced by in vitro organotypic assay when blocking ephrin-A5-binding ability with a soluble inhibitor (EphA7-Fc), arguing that type I SGNs express an appropriate EphA/EphB2 receptor needed to specifically interact with ephrin-A5. Differentially expressed among SGN populations, EphA4 was also found to be specifically activated through selective ephrin-A5-mediated type I growth cone collapse ( Fig. 5 ). In addition, forward signalling-deficient EphA4 EGFP/EGFP mice provide a radial shift in HC afferent innervation pattern comparable to the one observed in ephrin-A5 −/− animals. Given the crucial involvement of ephrin-A5/EphA4 interactions in establishing thalamocortical mapping [13] , we believe that, in the cochlea, the auditory innervation pattern is achieved on a similar model. Indeed, we show that EphA4 + type I SGNs connect ephrin-A5 − IHCs, whereas despite the presence of repulsive cues in target cells EphA4 − type II SGNs manage to project to ephrin-A5 + OHCs ( Fig. 7a and c ). Thus, it is tempting to speculate that EphA4 is the partner of ephrin-A5 in this repulsive/permissive system. In contrast, EphB2, although known to interact with ephrin-A5 [16] , does not seem to be a good candidate, as it is equally expressed in both type I and type II SGNs. 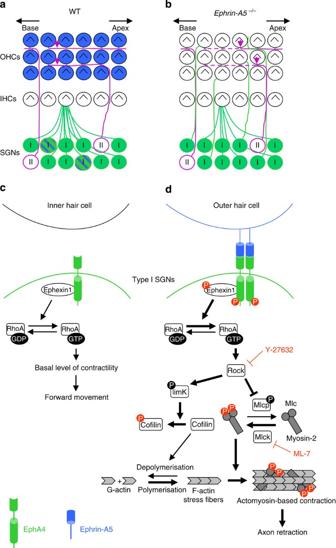Figure 7: Schematic model summarizing the contribution of ephrin-A5/EphA4 in afferent targeting to HCs in the OC. (a,b)Ephrin-A5(blue) andEphA4(green) genes are expressed at perinatal stages in OHCs and type I SGNs, respectively. These complementary patterns match one another given the known SG to HCs topography, with type I SGNs connecting IHCs and type II SGNs (purple) widely projecting to OHCs (purple arrowheads in A). (a) In the WT condition, ephrin-A5 from OHCs provides a repulsive signal to EphA4+type I axons (green). (b) In the absence ofephrin-A5, a subset of type I SGNs send ectopic projections to the OHCs region, giving rise to incomplete type II innervation (purple arrowheads indicate the new early endpoints) compared with WT (purple arrowheads in A). (c,d) A model for how ephrin-A5/EphA4 interactions control specific SGN afferent targeting to corresponding HCs. (c) When EphA4+type I SGNs reach ephrin-A5−IHCs, ephexin-1 is stably bound to EphA4 at the membrane, where it contributes to activation of RhoA, among other GTPases. RhoA supports a basal level of actomyosin-based contractility resulting in a forward movement. (d) When EphA4+type I SGNs reach ephrin-A5+OHCs, EphA4 activation enhances ephexin-1 activity toward RhoA. ROCK activation inhibits both cofilin-mediated f-actin depolymerization and myosin light chain phosphatase activity, favouring the accumulation of f-actin stress fibres and phospho-myosin light chain-2. Both components synergistically increase the actomyosin-based contraction, leading to growth cone collapse, therefore preventing type I SGN from targeting the OHCs. In red, the elements that were experimentally tested. limK, lim kinase; mlc, myosin light chain; mlcp, mlc phosphatase; mlck, mlc kinase. Figure 7: Schematic model summarizing the contribution of ephrin-A5/EphA4 in afferent targeting to HCs in the OC. ( a , b ) Ephrin-A5 (blue) and EphA4 (green) genes are expressed at perinatal stages in OHCs and type I SGNs, respectively. These complementary patterns match one another given the known SG to HCs topography, with type I SGNs connecting IHCs and type II SGNs (purple) widely projecting to OHCs (purple arrowheads in A). ( a ) In the WT condition, ephrin-A5 from OHCs provides a repulsive signal to EphA4 + type I axons (green). ( b ) In the absence of ephrin-A5 , a subset of type I SGNs send ectopic projections to the OHCs region, giving rise to incomplete type II innervation (purple arrowheads indicate the new early endpoints) compared with WT (purple arrowheads in A). ( c , d ) A model for how ephrin-A5/EphA4 interactions control specific SGN afferent targeting to corresponding HCs. ( c ) When EphA4 + type I SGNs reach ephrin-A5 − IHCs, ephexin-1 is stably bound to EphA4 at the membrane, where it contributes to activation of RhoA, among other GTPases. RhoA supports a basal level of actomyosin-based contractility resulting in a forward movement. ( d ) When EphA4 + type I SGNs reach ephrin-A5 + OHCs, EphA4 activation enhances ephexin-1 activity toward RhoA. ROCK activation inhibits both cofilin-mediated f-actin depolymerization and myosin light chain phosphatase activity, favouring the accumulation of f-actin stress fibres and phospho-myosin light chain-2. Both components synergistically increase the actomyosin-based contraction, leading to growth cone collapse, therefore preventing type I SGN from targeting the OHCs. In red, the elements that were experimentally tested. limK, lim kinase; mlc, myosin light chain; mlcp, mlc phosphatase; mlck, mlc kinase. Full size image This model is compatible with recent data showing that, during the anterior stage of fibre outgrowth and extension to the OC, EphA4 is expressed in the otic mesenchyme and interacts with ephrin-B2 on developing SGN axons [25] . Indeed, it can be suggested that, at late embryonic stages, EphA4 promotes SGN fasciculation through ephrin-B2 reverse signalling; once afferents have reached the OC, EphA4 (expressed in type I SGNs) forward signalling controls target specification through interaction with ephrin-A5 (expressed by OHCs) at early postnatal stages. Importantly, this hypothesis of a double role for EphA4 is supported by the fact that, in addition to be expressed in the otic mesenchyme, EphA4 mRNA was also found in the SG [25] . Perinatally, during HC innervation process, although type I fibres are specifically refined to basolateral regions of IHCs, some collateral branches (CBs) establish temporary synaptic contacts with OHCs that are pruned at later stages [5] , [37] , [38] . Importantly, numerous type I SGNs have both a main fibre refining to IHC and a CB forming a transient synapse with OHCs. How do these transient projections manage to reach ephrin-A5 + target cells? We observed that, in addition to be expressed in OHCs, ephrin-A5 seems to be dynamically expressed at perinatal stages in a subset of SGNs that do not belong to type II SGNs, therefore partially overlapping the expression of EphA4 ( Fig. 1o–u ). Although we found that this ephrin-A5 + SGN subpopulation reaches a peak at P0, knowing exactly whether this is a consistent subpopulation or whether type I SGNs are all expressing ephrin-A5 but at different times remains to be determined. Depending on the local neural network to be formed, recent work has shown that coexpressed Eph and ephrins cis -interact and mutually inactivate each other in the same cell, thereby fine-tuning the sensitivity of navigating axons to ephrins from the target tissue presented in trans [39] , [40] , [41] . Furthermore, the relative contribution of trans signalling and cis attenuation is influenced by the subcellular distribution of both ephrins and Ephs [39] , [42] . Therefore, it can be hypothesized that, within a given type I SGN in which EphA4 and ephrin-A5 are coexpressed, the presence of ephrin-A5 protein is exclusively confined to the CB, where it could mediate cis silencing of EphA4 forward signalling, preventing growth cone collapse and enabling the successful formation of transient type I—OHC synapses. By contrast, in the meantime, the main type I fibre would remain EphA4 + /ephrin-A5 − , involving the repulsion of type I fibre upon binding to ephrin-A5 + OHCs and the subsequent refinement to IHCs ( Supplementary Fig. 7 ). In WT condition, type II afferents enter the OHC area relatively apically, turn to the base, arborize extensively and innervate tens of cells. Although previous work supports the fact that neurite growth of type II SGNs is highly directed towards OHCs [43] , the mechanisms (neurotrophic or intrinsic) that would underlie this process remain largely unclear. Here we found that the absence of either ephrin-A5 or EphA4 forward signalling induces random invasion of the OHC layer by numerous ectopic fibres. Consequently, type II SGNs probably undergo axon competition and adapt by forming incomplete projections. This observation is consistent with the fact that competition for target territory refines the map by suppressing or eliminating branches [44] . Neuronal immunolabelings therefore reveal opposite shifts: a partial displacement of type I innervation from IHCs to OHCs and a subsequent withdrawal of type II projections from OHCs. This double defect is similar to what happens during retinocollicular map formation. Indeed, in the absence of ephrin-A5 anteroposterior gradient in the superior colliculus (SC) or EphA naso-temporal gradient in the retina, temporal axons (TAs) shift posteriorly. Nasal axons (NAs) therefore face increased competition in posterior SC, lose their affinity for this region and spread out anteriorly [14] , [45] . On the basis of gain- and loss-of-function analysis, a repulsion/competition model accounting for normal mapping has been proposed [14] , [46] . EphA + TAs are strongly repelled by posterior ephrins, and thus they terminate in the anterior SC. To avoid competition with TA in the anterior SC, EphA − NAs prefer to project only to the posterior SC. As similar defects were obtained in both situations using either ephrin-A5 −/− mice or in vivo loss of EphA function, such a model could be transposed from retinocollicular mapping to auditory projections pattern in the cochlea. EphA4 + type I fibres are repelled by ephrin-A5 from OHCs to IHCs. Founded on the observation that type II afferents fail to face strong type I axon competition in the OHC region, EphA4 − type II afferents could not compete against multiple and dense type I connections at IHCs and prefer to project to OHCs. Such an explanation is not far from the idea that type I afferents may reach the OC earlier and occupy the available membrane surface on IHCs, thus leaving free synaptic space only on OHCs for type II fibers [37] . To precisely address this competition hypothesis, a mouse line devoid of type I SGNs should be created in order to observe whether, in the absence of competition, some type II SGNs connect the IHCs. Electrophysiological measurements revealed that ephrin-A5 is dispensable for a normal hearing threshold. Given that type I afferents initially indifferently reach both types of HCs [5] , in the absence of ephrin-A5 , a subset of type I projections should directly connect IHCs without interacting with OHCs. This residual type I innervation persisting at IHCs ( Fig. 2 ) would therefore be sufficient to preserve a normal hearing threshold. However, an impaired neurotransmission from IHCs to the auditory nerve was recorded in ephrin-A5 −/− animals and should result from the partial type I SGN mistargeting to OHCs, leading to the lack of IHC—type I afferent synapses. Interestingly, EphA4 − / − mice show a similar decrease of ABR peak 1 amplitude [47] , reinforcing the hypothesis of a complementary contribution to ephrin-A5 in specific afferent targeting to HCs. Ribbon quantification revealed that radial shift of type I projections from IHCs to OHCs in both ephrin-A5 −/− and EphA4 EGFP/EGFP mice is accompanied by an increased number of presynaptic active zones in the OHC area ( Figs 2and 4 ). During the first postnatal week, type I SGNs extend transient collateral projections to OHCs [5] and form synapses that express glutamate receptor subtypes [48] and trigger Ca 2+ - and otoferlin-dependent glutamate release, similar to what occurs in mature IHCs [49] . In adult cochlea, ribbons are believed to support afferent signalling from OHCs [50] . Concurrently, these findings suggest the idea that, in either ephrin-A5 −/− or EphA4 forward signalling-deficient mice, some definitive type I—OHC ribbon-containing synapses could enhance the afferent neurotransmission from this region. Altogether, our results indicate that, rather than occurring by any mechanisms of specific attraction as initially suggested [35] , the precise targeting of type I SGNs—IHCs versus type II SGNs—OHCs is dependent on ephrin-mediated mutual repulsion through matching complementary expression patterns of ephrin and Eph genes. This crucial finding could be usefully exploited in therapeutic strategies aimed at improving the neurotransmission from HCs to the cochlear nerve by selectively optimizing the afferent innervation of either IHCs or OHCs. Animals WT and ephrin-A5 −/− , EphA4 +/EGFP and EphA4 EGFP/EGFP littermates were obtained from heterozygous crosses, and the genotype was determined by PCR as previously described [9] , [26] . Mice were group-housed in the animal facility of the University of Liège under standard conditions with food and water ad libitum and were maintained on a 12-h light/dark cycle. All animals were taken care of in accordance with the declaration of Helsinki and following the guidelines of the Belgian ministry of agriculture in agreement with EC laboratory animal care and use regulation (86/609/CEE, CE of J n°L358, 18 December 1986). In vitro organotypic assay SG and OC were isolated together from E18 mouse cochleae and cultured in DMEM (Gibco) supplemented with glucose (final concentration 6 g l −1 ) and N1 additives (insulin (5 μg ml −1 ), transferrin (5 μg ml −1 ), putrescin (10 − 4 M), progesterone (2 × 10 − 8 M) and selenium ([Na 2 SeO 3 ] 3 × 10 − 8 M)). Explants were treated with either IgG-Fc fragment as control or recombinant mouse EphA7-Fc chimera (5 μg ml −1 ; R&D Systems, Minneapolis, MN, USA), an ephrin-A5 inhibitor, during 4 days. Explants were also treated during the same time window with dimethylsulphoxide as control or Y-27632 dihydrochloride (10 μM; Tocris, Bristol, UK), a selective inhibitor of the RhoA-associated protein kinase p160ROCK and ML-7 (10 μM; Sigma-Aldrich, St Louis, MO, USA), a selective MLCK inhibitor. Primary culture of SGNs and growth cone collapse assay SGNs from newborn mice were isolated, cultured as previously described [51] and incubated with a 5 μg ml −1 human ephrin-A5-Fc (R&D systems, Minneapolis, MN, USA) solution pre-clustered for 1 h at 37 °C with 50 μg ml −1 anti-human IgG-Fc (R&D systems, Minneapolis, MN, USA). Before beginning growth cone collapse assay, cells were pre-treated with either Y-27632 dihydrochloride (7 h, 10 μM; Tocris, Bristol, UK) or ML-7 (5 h, 10 μM; Sigma-Aldrich, St Louis, MO, USA). After incubation with pre-clustered ephrin-A5 for 15 min in a humidified atmosphere of 5% CO 2 /95% air, SGNs were then fixed in 4% paraformaldehyde and immunolabeled using peripherin (rabbit polyclonal antibody, 1:100; Santa Cruz Biotechnology, Santa Cruz, CA, USA), EphA4 (tyr-602) phospho-specific (rabbit polyclonal antibody, 1:100; ECM Biosciences, Versailles, KY, USA), green fluorescent protein (rat monoclonal IgG2a, 1:100; Gentaur, London, UK), ephexin-1 (tyr-87) phospho-specific (rabbit polyclonal antibody, 1:100; ECM Biosciences, Versailles, KY, USA), phospho-myosin light chain 2 (ser-19) (rabbit polyclonal antibody, 1:100; Cell Signaling, Danvers, MA, USA) or phospho-cofilin (ser-3) (rabbit monoclonal antibody, 1:100; Cell Signaling, Danvers, MA, USA) antibodies and tetramethyl rhodamine isothiocyanate-phalloidin (1:500; Sigma-Aldrich, St Louis, MO, USA) as an F-actin marker. The criteria for collapsed growth cones were a total loss of filopodia and lamellipodia and a strong decrease in F-actin content. Data were statistically analysed using one-way analysis of variance (ANOVA) followed by a Dunnett’s post-test (GraphPad Prism software 4.0; GraphPad Software Inc., San Diego, CA, USA). P- values <0.05 were considered significant (** P <0.01). Tissue processing and immunostainings Embryo heads and postnatal cochleae were fixed for 2–24 h (time according to the sample size) in 4% paraformaldehyde and, if needed, decalcified for at least three days (0.1 M EDTA in PBS). Whole-mount cochleae, sections or explants were incubated overnight at 4 °C with primary antibodies directed against ephrin-A5 (goat IgG, 1:100; Santa Cruz Biotechnology, Santa Cruz, CA, USA), green fluorescent protein (rat monoclonal IgG2a, 1:250; Gentaur, London, UK), peripherin (mouse monoclonal IgG1, 1:250; Acris Antibodies GmbH, Herford, Germany), βIII-tubulin (Tuj1 antibody, mouse monoclonal IgG2a, 1:2000; Covance Reaserch Products, Princeton, NJ, USA), myosin-VII (rabbit IgG, 1:250; Santa Cruz Biotechnology, Santa Cruz, CA, USA) and parvalbumin (goat IgG, 1:5000; Swant, Marly, Switzerland), both specific markers for HCs [52] , [53] , neurofilament H (rat IgG, clone TA51, 1:500; Millipore, Billerica, MA, USA) and CtBP2/RIBEYE (purified mouse IgG1, 1:250; BD Transduction Laboratories, Mississauga, ON, Canada). Tissues were then incubated for 1 h with either Rhodamine Red X-, fluorescein isothiocyanate- or Cy5-conjugated goat anti-mouse, anti-rabbit or anti-rat IgGs secondary antibodies (Jackson Immunoresearch Laboratories, Suffolk, UK). For glutamate receptor subunit 2/3 (rabbit IgG, 1:200; Chemicon, Temecula, CA, USA)/CtBP2 double immunolabeling, freshly dissected apical cochlear turns were fixed with 99.9% ethanol (Merck, Darmstadt, Germany) for 20 min at −20 °C. Confocal microscopy, image analysis and quantifications Fluorescence pictures were acquired using the Olympus Fluoview FV1000 confocal system equipped with the Olympus IX81 inverted microscope (Olympus Europa GmbH, Germany) or the Leica SP2 confocal microscope (Leica, Wetzlar, Germany). Unless otherwise mentioned, fields were acquired using Z-scan, with a step of 1 μm between each confocal plane. For comparison between genotypes and culture conditions, all preparations were analysed at the same time, using the same acquisition parameters. On whole-mount P2, 3-month and P14 cochleae, we considered, respectively, the proportion of NF-H + fibres beneath and beyond the row of IHCs and the number NF-H + /peripherin – fibres between IHC and OHC layers. Each explant was cut into three fragments consisting of apical, middle and basal turns of cochleae from WT, ephrin-A5 −/− and EphA4 EGFP/EGFP mice, and one corresponding region (as shown, for the apical turn, in Fig. 2a (magnifications)) measuring roughly 200 μm was considered for quantification. To avoid multiplication of graphs and statistics, in each case, data from individual turns were collapsed to give a single cochlea figure. At P2 and at 3 months, values were expressed as a percentage of fibres targeting the OHC layer. At P14, values were expressed as a mean axon number per 100 μm of cochlear length for each animal. Data were statistically analysed using a Student’s t -test. P- values <0.05 were considered significant (** P <0.01; *** P <0.001). On whole-mount P14 cochleae, type II fibres were classified in two groups of length <200 or >200 μm after entering the OC. Measures were done using ImageJ software (NIH). Data were statistically analysed using Student’s t -test. P- values <0.05 were considered significant (* P <0.05; ** P <0.01). For each organotypic culture condition, we compared the number of βIII-tubulin + fibres beneath and beyond the row of IHCs, and values were expressed as a percentage of fibres targeting the OHC layer. Depending on the number of conditions to be compared, data were statistically analysed using a Student’s t -test or a one-way ANOVA test followed by a Dunnett’s post-test. P- values <0.05 were considered significant (** P <0.01; *** P <0.001). CtBP2 + synaptic ribbons were quantified in about 12–15 IHCs and corresponding tangential OHCs in similar regions from apical, middle and basal turns of P14 cochleae from WT and ephrin-A5 −/− or EphA4 EGFP/EGFP mice. The number of ribbons was divided by the total number of IHC nuclei to obtain the number of synaptic ribbons/IHC or/row of OHCs (classically corresponding to three OHCs). In a subset of cochleae in which co-labelling for ribbons and postsynaptic AMPA receptors was performed, juxtaposed spots of ribbon and AMPA receptor immunofluorescence were counted and expressed as the number of synapses per IHC. Data were statistically analysed using a Student’s t -test. P- values <0.05 were considered significant (* P <0.05; ** P <0.01; *** P <0.001). Total SGNs and type II SGNs from WT, ephrin-A5 −/− or EphA4 EGFP/EGFP P2 mice were quantified using a stereological reconstruction method [54] . Data were statistically analysed using a Student’s t -test. In organotypic cultures, SGN population was quantified by considering three fields of SG per condition. Values were expressed as a mean number of SGNs per 10000 μm 2 . Depending on the number of conditions to be compared, data were statistically analysed using a Student’s t -test or a one-way ANOVA test. Ephrin-A5 + and EphA4 + SGNs were quantified at apical, middle and basal turns of E18—P6 cochleae after in situ hybridization (ISH) and βIII-tubulin immunolabeling. Roughly 500 SGNs were quantified for each animal and for each probe. Data were expressed as a percentage of SGNs expressing ephrin-A5 or EphA4 . RNA ISH ISH was performed using digoxigenin-labelled ephrin-A5 (ref. 55 ) and EphA4 (ref. 56 ) riboprobes as previously described [57] . If needed, slides were classically immunolabeled with peripherin or βIII-tubulin antibodies. In vitro stripe assay Stripe assay using recombinant control IgG-Fc or pre-clustered ephrin-A5-Fc was performed as previously described [58] . Ephrin-A5 stripes were labelled using anti-human IgG (Fc-specific)-Cy3-conjugated antibodies (1:100; Sigma-Aldrich, St. Louis, MO, USA). SGs from newborn mice were dissected and plated on stripes for 24–48 h. Neurons were then labelled using Calcein AM (1:1000; Invitrogen Molecular Probes, Eugene, OR, USA) for 1 h at 37 °C, and pictures were acquired using the Olympus Fluoview FV1000 confocal system. Data were analysed by comparing the percentage of growth cones present in control IgG-Fc or ephrin-A5-Fc stripes using a Student’s t -test. P- value <0.05 was considered significant (** P <0.01). ABR recording Three-month-old mice were recorded as previously described [59] . ABR threshold was determined by detection of any wave in the complex. Data were statistically analysed using a Student’s t -test. P- values <0.05 were considered significant (* P <0.05; ** P <0.01). How to cite this article: Defourny, J. et al . Ephrin-A5/EphA4 signalling controls specific afferent targeting to cochlear hair cells. Nat. Commun. 4:1438 doi: 10.1038/ncomms2445 (2013).